Phosphatidylinositol-3-phosphate regulates sorting and processing of amyloid precursor protein through the endosomal system Defects in endosomal sorting have been implicated in Alzheimer’s disease. Endosomal traffic is largely controlled by phosphatidylinositol-3-phosphate, a phosphoinositide synthesized primarily by lipid kinase Vps34. Here we show that phosphatidylinositol-3-phosphate is selectively deficient in brain tissue from humans with Alzheimer’s disease and Alzheimer’s disease mouse models. Silencing Vps34 causes an enlargement of neuronal endosomes, enhances the amyloidogenic processing of amyloid precursor protein in these organelles and reduces amyloid precursor protein sorting to intraluminal vesicles. This trafficking phenotype is recapitulated by silencing components of the ESCRT (Endosomal Sorting Complex Required for Transport) pathway, including the phosphatidylinositol-3-phosphate effector Hrs and Tsg101. Amyloid precursor protein is ubiquitinated, and interfering with this process by targeted mutagenesis alters sorting of amyloid precursor protein to the intraluminal vesicles of endosomes and enhances amyloid-beta peptide generation. In addition to establishing phosphatidylinositol-3-phosphate deficiency as a contributing factor in Alzheimer’s disease, these results clarify the mechanisms of amyloid precursor protein trafficking through the endosomal system in normal and pathological states. Alzheimer’s disease (AD) is the most common neurodegenerative disorder and is characterized by a progressive decline in cognitive function [1] , [2] , [3] . Brain regions affected by AD display neuronal loss as well as amyloid plaques and neurofibrillary tangles. Amyloid plaques largely consist of the amyloid-β (Aβ) peptide, which is released by cleavage of amyloid precursor protein (APP) by the β-secretase Beta-site APP cleavage enzyme 1 (BACE1) and γ-secretase. Autosomal dominant mutations in the genes encoding APP and presenilins 1 and 2, the proteases of the γ-secretase complex, lead to rare early-onset familial cases of AD (FAD). In contrast, the majority of AD cases occur later in life (that is, late-onset AD or LOAD) with no precise cause, although an allelic variant of the gene-encoding apolipoprotein E, ApoE4, has been identified as a major risk factor [3] . Overall, the molecular and cellular mechanisms underlying LOAD are poorly understood. APP traffics through organelles of the biosynthetic, secretory and endolysosomal pathways, and undergoes differential and compartment-specific processing by α-, β- and γ-secretases [1] , [4] . Several converging lines of evidence indicate that the amyloidogenic cleavage of APP occurs predominantly in endosomes [4] , [5] . First, the proteolytic activity of BACE1 is optimal at a mildly acidic pH, making the endosomal environment ideal for β-secretase-mediated cleavage of APP [6] . Second, APP appears to interact with BACE1 primarily in the endocytic pathway [4] , [7] , [8] , [9] . Third, reducing the access of APP or BACE1 to endosomes by blocking their internalization via clathrin or the small GTPase Arf6, respectively, decreases the amyloidogenic processing of APP [4] , [9] , [10] , [11] , [12] , [13] , [14] . Fourth, β-cleaved COOH-terminal fragments (CTFs) of APP have been shown to be produced in endosomes [15] , where they can be further processed by γ-secretase [16] . Consistent with all these observations, various studies have documented abnormal endosomal morphology and increased endosomal Aβ burden in the brain of individuals with AD, suggesting that endosomal dysfunction may be the key to AD pathogenesis [5] , [17] , [18] , [19] . Importantly, expression studies have identified LOAD-associated deficiencies in a range of molecules related to the retromer pathway, which regulates the sorting of transmembrane proteins from endosomes to the trans -Golgi network (TGN) or the cell surface [20] , [21] , [22] . These include retromer components (Vps26, Vps29, Vps35) and retromer receptors (SorL1 and SorCS1), which have been implicated in APP sorting and processing [1] , [21] , [22] , [23] . Finally, neurons derived from the fibroblasts of patients with presenilin mutations [24] , APP duplications or LOAD [25] show an enlargement of early endosomes. Thus, endosomal dysfunction is increasingly viewed as a key cellular phenotype of AD. A master organizer of endosomal sorting is the signalling phosphoinositide phosphatidylinositol-3-phosphate (PI3P) [26] , [27] , which acts by recruiting to endosomal membranes a variety of effectors containing PI3P-binding modules, such as PX (Phox homology) and FYVE (Fab1, YOTB, Vac1, EEA1) domains [27] . These effectors control trafficking aspects as diverse as the budding of retromer-coated tubules (for example, SNX1,2,6,27), the fusion of endosomes (for example, EEA1) and the ESCRT-dependent intraluminal sorting of ubiquitinated cargos in multivesicular endosomes (for example, Hrs). A major pathway for the synthesis of PI3P involves class III PI 3-kinase Vps34, which phosphorylates PI on the 3′-position of the inositol ring [27] . Disrupting the function of Vps34 through various approaches causes pleiotropic defects in endosomal function [27] . Finally, PI3P controls macroautophagy, and regulators of this degradative pathway such as beclin1 act in part through a modulation of Vps34 and show decreased levels in brain from LOAD patients [28] , [29] . As AD pathogenesis is linked to endosomal anomalies, we hypothesized that a perturbation of PI3P metabolism may occur in brain regions most affected by the disease, and that this disruption could contribute to pathogenic processes. Our study shows a selective PI3P deficiency in the prefrontal cortex (PFC) and entorhinal cortex (ERC) of LOAD-affected individuals as well as in FAD mouse models. We further show that silencing Vps34, and thus reducing PI3P levels, recapitulates several features of AD, including endosomal anomalies and enhanced amyloidogenic processing of APP. In addition, we establish that APP is both ubiquitinated and sorted into endosomal intraluminal vesicles (ILVs) via the PI3P-dependent ESCRT pathway, with major implications for its metabolism. Together, our results identify the PI3P–ESCRT pathway as a novel contributing factor in APP biology and potentially, AD pathogenesis. PI3P levels are decreased in AD-affected brains To test whether PI3P levels are aberrant in brain regions affected with LOAD, we optimized the high-performance liquid chromatography-mediated separation of PI3P and PI4P and were able to detect and quantify these two lipids using suppressed conductivity [30] , [31] ( Supplementary Fig. S1 ). Brain regions affected in the AD (PFC and ERC) or relatively spared (cerebellum (CRB)) were analysed. Although PI4P levels were unchanged, a deficiency of PI(4,5)P 2 was observed in the PFC of AD patients, consistent with our studies showing that the metabolism of this lipid is disrupted by Aβ, particularly at synapses [31] , [32] . Importantly, a significant decrease in PI3P was found in PFC (~40%) and, to a lower extent, ERC (~25%), but not in the CRB from AD patients ( Fig. 1a ). PI3P levels were also measured in the forebrain of three commonly used transgenic mouse models of familial AD (FAD), namely, (i) PSEN1 M146V (PS), (ii) the Swedish mutant of APP K670N,M671L (APP) and (iii) PS-APP double transgenic lines [33] . We found a selective decrease in PI3P levels in each of the mouse model of FAD (that is, an ~25% decrease in the APP and PS1 models and an ~40% decrease in the PS1-APP model; Fig. 1b ). Importantly, when the phosphoinositide data was combined with a recent mass spectrometry-based lipidomic analysis of the same samples [33] and expressed as a heat map, the PI3P deficiency was the only lipid alteration common to both human and mouse brain affected with AD out of ~330 lipid species and 29 lipid classes ( Fig. 1c ). These data indicate that the deficiency of PI3P observed in both LOAD- and FAD-affected brains is highly selective. 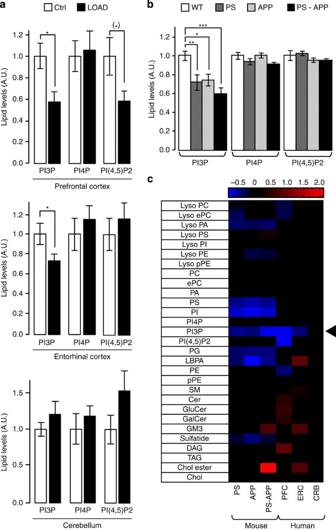Figure 1: PI3P levels are decreased in the human and mouse brain affected by AD. (a) Bar diagram showing relative phosphoinositide levels in the PFC, ERC and CRB from post-mortem brains of either non-AD human subjects (ctrl) or late-onset AD human subjects (LOAD). Measurements were made by anionic exchange high-performance liquid chromatography (HPLC) with suppressed conductivity detection and expressed in arbitrary units, relative to control levels. Values are shown as means±s.e.m. (PFC, ctrln=10 and LOADn=10; ERC and CRB, ctrln=12 and LOADn=15). The PI(4,5)P2deficiency in the PFC was significant (P<0.05) with a one-tailed Student’st-test and is indicated by (*) (see Methods). Otherwise, *P-values<0.05 using one-way analysis of variance (ANOVA) withpost hocTukey test. (b) Bar diagram showing relative phosphoinositide levels in the forebrain of FAD mouse models. These include the PSEN1M146V(PS), the Swedish mutant of APPK670N,M671L(APP) and the PS-APP double transgenic lines. Measurements were made by anionic exchange HPLC with suppressed conductivity detection and expressed in arbitrary units, relative to control levels. Values are shown as means±s.e.m. (n=6). *, ** and ***P-values<0.05, 0.01 and 0.001, respectively, using one-way ANOVA withpost hocTukey test. (c) Heat map showing all lipid classes measured and organized according to phospholipids, sphingolipids and neutral lipids classification. The PS, APP, PS-APP columns represent the normalized values of the individual lipid species of mutant mice compared with wild-type mice, whereas the PFC, ERC and CRB columns represent the normalized values of the individual lipid species of LOAD patients compared with control patients for each tissue type. The colour bars represents the log2 value of the ratio of each lipid species and only statistically significant changes are shown (P<0.05). PFC, ctrln=10 and LOADn=10; ERC and CRB, ctrln=12 and LOADn=15. The arrowhead indicates the PI3P change. Figure 1: PI3P levels are decreased in the human and mouse brain affected by AD. ( a ) Bar diagram showing relative phosphoinositide levels in the PFC, ERC and CRB from post-mortem brains of either non-AD human subjects (ctrl) or late-onset AD human subjects (LOAD). Measurements were made by anionic exchange high-performance liquid chromatography (HPLC) with suppressed conductivity detection and expressed in arbitrary units, relative to control levels. Values are shown as means±s.e.m. (PFC, ctrl n =10 and LOAD n =10; ERC and CRB, ctrl n =12 and LOAD n =15). The PI(4,5)P 2 deficiency in the PFC was significant ( P <0.05) with a one-tailed Student’s t -test and is indicated by (*) (see Methods). Otherwise, * P -values<0.05 using one-way analysis of variance (ANOVA) with post hoc Tukey test. ( b ) Bar diagram showing relative phosphoinositide levels in the forebrain of FAD mouse models. These include the PSEN1 M146V (PS), the Swedish mutant of APP K670N,M671L (APP) and the PS-APP double transgenic lines. Measurements were made by anionic exchange HPLC with suppressed conductivity detection and expressed in arbitrary units, relative to control levels. Values are shown as means±s.e.m. ( n =6). *, ** and *** P -values<0.05, 0.01 and 0.001, respectively, using one-way ANOVA with post hoc Tukey test. ( c ) Heat map showing all lipid classes measured and organized according to phospholipids, sphingolipids and neutral lipids classification. The PS, APP, PS-APP columns represent the normalized values of the individual lipid species of mutant mice compared with wild-type mice, whereas the PFC, ERC and CRB columns represent the normalized values of the individual lipid species of LOAD patients compared with control patients for each tissue type. The colour bars represents the log2 value of the ratio of each lipid species and only statistically significant changes are shown ( P <0.05). PFC, ctrl n =10 and LOAD n =10; ERC and CRB, ctrl n =12 and LOAD n =15. The arrowhead indicates the PI3P change. Full size image APP is found on PI3P- and Vps34-positive endosomes We next investigated the relationship between APP, Vps34 and its product PI3P using confocal microscopy. Attempts to localize endogenous Vps34 were unsuccessful because of the lack of specific antibodies, so HeLa cells were transfected with tagged constructs of Vps34 (Vps34 RFP ), APP (APP myc ) and a genetically encoded probe for PI3P, that is, the tandem FYVE domain of EEA1 (FYVE-FYVE GFP ) [34] . We found that the majority of APP immunoreactivity localizes to Vps34 RFP - and PI3P-positive structures ( Supplementary Fig. S2a ), consistent with their predominant localization in endosomes. Both Vps34 RFP and APP myc colocalized with endogenous markers of early (EEA1) and, to a lesser extent, late (LAMP1) endosomal compartments ( Supplementary Figs S2b and S3a,b ). Of note, although ~65% of APP colocalizes with EEA1, a smaller pool (~35%) is found in the late Golgi, as revealed by an anti-giantin staining ( Supplementary Fig. S2b ), consistent with previous literature (see for instance ref. 35 ). Not only full-length APP, but also its CTFs were found to be enriched in endosomes obtained by subcellular fractionation of HeLa cell extracts ( Supplementary Fig. S3c ), suggesting extensive processing of APP in these organelles. Finally, because Vps34 has been implicated in autophagosome formation and maturation [29] and that APP processing can also occur in these structures [36] , we examined the localization of APP RFP and the autophagosomal marker LC3 upon starvation and found no colocalization ( Supplementary Fig. S3d ), suggesting that APP RFP does not traffic through autophagosomes, at least under these conditions. Together, these data show a tight association between APP and the Vps34- and PI3P-positive endosomes. Silencing Vps34 enhances amyloidogenic processing of APP We next investigated the impact of PI3P deficiency on the processing of endogenous APP. Lentiviruses expressing short hairpin RNAs against murine Vps34 (shVps34) or control short hairpin RNAs (shRNAs) (shCTRL) were used to infect mature primary cortical neurons for 7 days. Aβ40 and Aβ42 levels were subsequently analysed in media. In the shVps34 conditions ( Fig. 2a ), levels of Aβ42 and Aβ40 peptides were each increased by ~2-fold ( Fig. 2b ), with no change in the Aβ42/Aβ40 ratio ( Fig. 2c ). Full-length APP showed a trend for an increase ( Fig. 2a ), although the APP messenger RNA was not upregulated (1.007±0.002 for the shVps34 condition compared with 1.000±0.318 for the shMock condition, in normalized units, P >0.05). Levels of the secreted fragment of APP produced by α-secretase (sAPP-α) were not affected by shVps34, although a trend for an increase in the levels of the secreted fragment of APP produced by β-secretase (sAPP-β) was observed (Fig. 2d ). Unfortunately, endogenous APP CTFs were not detectable. Importantly, silencing Vps34 produced an ~45% increase in the size of EEA1-positive endosomal puncta ( Fig. 2e ), consistent with previous studies [37] . Together, these data demonstrate that a deficiency of Vps34 causes endosomal abnormalities and enhances the amyloidogenic processing of APP in neurons, establishing a link between PI3P deficiency, endosomal dysfunction and AD pathogenesis. 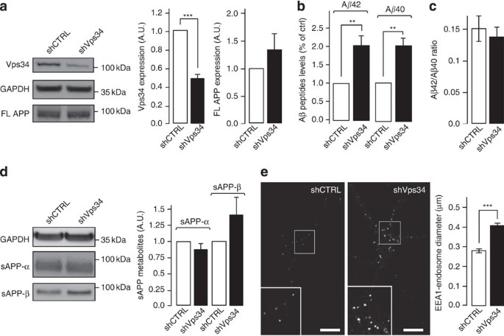Figure 2: Silencing of Vps34 leads to increased amyloidogenic processing of neuronal APP. (a) Western blot analysis (left panel) of endogenous Vps34 and full-length APP (FL-APP) levels in cultured mouse cortical neurons infected with Vps34-shRNA lentivirus (shVps34) or a control lentivirus (shCTRL). GAPDH was used as an equal loading marker. The graphs show the quantification of Vps34 levels (middle panel) and FL-APP levels (right panel) in arbitrary units. Values denote means±s.e.m. (n=17). ***P-values<0.001 using Student’st-test. (b) Bar diagram showing murine Aβ42 and Aβ40 levels measured by enzyme-linked immunosorbent assay (ELISA) from cultured cortical neuron media, after infection with shCTRL or shVps34 lentiviruses. Aβ levels were normalized to the cell lysate total protein. Values are shown as means±s.e.m. (n=13). **P-values<0.01 using Student’st-test. (c) Bar diagram showing the Aβ42/Aβ40 ratio measured from experiments described inband is shown as means±s.e.m. (n=13). (d) Quantification of secreted APP metabolites derived from the cleavage of murine sAPP-α or sAPP-β after infection of cultured cortical neurons with shCTRL or shVps34 lentiviruses. Left panel, western blot analysis of secreted fragments in the media alongside the loading control GAPDH. Right panel, bar diagram showing the quantification of sAPP-α (left bars) and sAPP-β levels (right bars) after normalization of their levels to the cell lysate total protein. Values denote means±s.e.m. (sAPP-αn=7, sAPP-βn=5). (e) Confocal analysis of cultured mouse cortical neurons infected with shCTRL or shVps34 lentiviruses and stained with an EEA1-specific antibody. Left panel, representative immunostainings. Scale bar, 10 μm. Right panel, bar diagram showing the average diameter of EEA1-positive endosomal fluorescent puncta. Values denote means±s.e.m. (n=82). ***P-values<0.001 using Student’st-test. Figure 2: Silencing of Vps34 leads to increased amyloidogenic processing of neuronal APP. ( a ) Western blot analysis (left panel) of endogenous Vps34 and full-length APP (FL-APP) levels in cultured mouse cortical neurons infected with Vps34-shRNA lentivirus (shVps34) or a control lentivirus (shCTRL). GAPDH was used as an equal loading marker. The graphs show the quantification of Vps34 levels (middle panel) and FL-APP levels (right panel) in arbitrary units. Values denote means±s.e.m. ( n =17). *** P -values<0.001 using Student’s t -test. ( b ) Bar diagram showing murine Aβ42 and Aβ40 levels measured by enzyme-linked immunosorbent assay (ELISA) from cultured cortical neuron media, after infection with shCTRL or shVps34 lentiviruses. Aβ levels were normalized to the cell lysate total protein. Values are shown as means±s.e.m. ( n =13). ** P -values<0.01 using Student’s t -test. ( c ) Bar diagram showing the Aβ42/Aβ40 ratio measured from experiments described in b and is shown as means±s.e.m. ( n =13). ( d ) Quantification of secreted APP metabolites derived from the cleavage of murine sAPP-α or sAPP-β after infection of cultured cortical neurons with shCTRL or shVps34 lentiviruses. Left panel, western blot analysis of secreted fragments in the media alongside the loading control GAPDH. Right panel, bar diagram showing the quantification of sAPP-α (left bars) and sAPP-β levels (right bars) after normalization of their levels to the cell lysate total protein. Values denote means±s.e.m. (sAPP-α n =7, sAPP-β n =5). ( e ) Confocal analysis of cultured mouse cortical neurons infected with shCTRL or shVps34 lentiviruses and stained with an EEA1-specific antibody. Left panel, representative immunostainings. Scale bar, 10 μm. Right panel, bar diagram showing the average diameter of EEA1-positive endosomal fluorescent puncta. Values denote means±s.e.m. ( n =82). *** P -values<0.001 using Student’s t -test. Full size image Silencing Vps34 perturbs APP trafficking To test whether silencing Vps34 perturbs the endosomal localization of APP, we conducted confocal analyses of primary neurons immunostained with antibodies to the cytodomain of endogenous APP as well as to EEA1 and GM130 to label the endosomal and Golgi compartments, respectively ( Fig. 3a,b ). Silencing Vps34 produced a major loss of APP fluorescence from EEA1-positive endosomes ( Fig. 3c ) and an apparent and relative increase in the Golgi compartment, which primarily reflects the loss of endosomal fluorescence ( Fig. 3d ). As γ-secretase releases the cytodomain of APP in the cytosol, loss of the APP cytodomain immunoreactivity from endosomes may reflect increased processing of APP CTFs by γ-secretase because of Vps34 silencing. To test this, neurons infected with the shCTRL or shVps34 lentiviruses were treated with vehicle or a γ-secretase inhibitor, compound XXI. Although the γ-secretase inhibitor did not affect the localization of APP in shCTRL-treated neurons, it fully restored the normal distribution of APP in shVps34-treated neurons ( Fig. 3c,d ). These data suggest that the increased processing of APP occurring upon silencing of Vps34 primarily takes place in endosomes (although minor contributions from the Golgi cannot be excluded) and prompted us to investigate the precise role of this enzyme and its product PI3P in the endosomal sorting of APP. 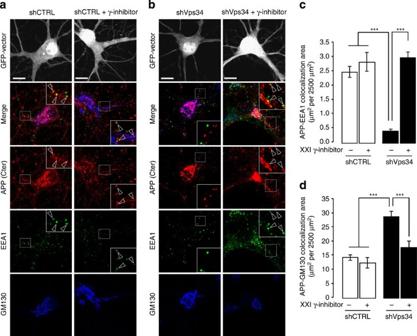Figure 3: Silencing of Vps34 alters the subcellular localization and processing of endogenous APP. (a) Mouse hippocampal neurons were transfected with shCTRLGFPplasmid at DIV 8 and cultured for 3 days before a 24-h treatment with vehicle (left panel) or γ-secretase inhibitor compound XXI at 10 μM (right panel). Neurons were then fixed, stained for the indicated antibodies (anti-GM130, blue channel, anti-EEA1, green channel and anti-APP COOH-terminus (C-term) antibody, red channel) and imaged using confocal microscopy. Scale bar, 10 μm. Arrowheads indicate structures showing colocalization between APP and EEA1. (b) Mouse hippocampal neurons were transfected with shVps34GFPand processed as described ina. (c) Bar diagram showing the amount of colocalization between APP and EEA1 per 2500 μm2of image cell surface area following expression of shCTRLGFP(seea) or shVps34GFP(seeb) in cultured neurons, in the presence or absence of γ-secretase inhibitor XXI. Results are shown as means±s.e.m. (n=30 cells). ***P-values<0.001 using Student’st-test. (d) Bar diagram showing the amount of colocalization between APP and GM130 per 2500 μm2of image cell surface area following expression of shCTRLGFP(seea) or shVps34GFP(seeb) in cultured neurons, in the presence or absence of γ-secretase inhibitor XXI. Results are shown as means±s.e.m. (n=28 cells). ***P-values<0.001 using Student’st-test. Figure 3: Silencing of Vps34 alters the subcellular localization and processing of endogenous APP. ( a ) Mouse hippocampal neurons were transfected with shCTRL GFP plasmid at DIV 8 and cultured for 3 days before a 24-h treatment with vehicle (left panel) or γ-secretase inhibitor compound XXI at 10 μM (right panel). Neurons were then fixed, stained for the indicated antibodies (anti-GM130, blue channel, anti-EEA1, green channel and anti-APP COOH-terminus (C-term) antibody, red channel) and imaged using confocal microscopy. Scale bar, 10 μm. Arrowheads indicate structures showing colocalization between APP and EEA1. ( b ) Mouse hippocampal neurons were transfected with shVps34 GFP and processed as described in a . ( c ) Bar diagram showing the amount of colocalization between APP and EEA1 per 2500 μm 2 of image cell surface area following expression of shCTRL GFP (see a ) or shVps34 GFP (see b ) in cultured neurons, in the presence or absence of γ-secretase inhibitor XXI. Results are shown as means±s.e.m. ( n =30 cells). *** P -values<0.001 using Student’s t -test. ( d ) Bar diagram showing the amount of colocalization between APP and GM130 per 2500 μm 2 of image cell surface area following expression of shCTRL GFP (see a ) or shVps34 GFP (see b ) in cultured neurons, in the presence or absence of γ-secretase inhibitor XXI. Results are shown as means±s.e.m. ( n =28 cells). *** P -values<0.001 using Student’s t -test. Full size image APP is sorted into the ILVs of multivesicular endosomes A key function of Vps34 and PI3P is to control the sorting of cargos into ILVs of multivesicular endosomes via the ESCRT pathway, which typically ensures their degradation in lysosomes [38] , [39] . We thus tested whether aberrant processing of APP caused by Vps34 deficiency reflects a contribution of this pathway. To begin to address this issue, we attempted to visualize intraluminal APP in HeLa cells using confocal microscopy, following expression of APP RFP and the constitutively active form of Rab5, Rab5 Q79L GFP , which is locked in its GTP-bound form [15] , [40] . This mutant is known to produce an enlargement of endosomes, allowing for the discrimination between the limiting membrane of these organelles and their lumen, which contains the ILVs. Under these conditions, APP RFP , and probably CTFs thereof, were mostly observed within the endosomal lumen, in contrast to endosomal markers known to be associated with the limiting membrane, including Rab5 itself, EEA1, or the retromer component Vps35 ( Fig. 4a ). Analysis of APP RFP - and Rab5 Q79L GFP -positive endosomes showed that ~70% of these structures display luminal fluorescence, probably reflecting an association of APP RFP with ILVs ( Fig. 4b ). Comparable results were obtained with the CTF-β (data not shown; see also ref. 15 ). Immunoelectron microscopic (EM) analysis of APP GFP using anti-green fluorescent protein (GFP) antibodies showed gold particles inside multivesicular structures, confirming the light microscopic observations ( Supplementary Fig. S4a ). Importantly, endogenous APP was also predominantly found (~80%) in the lumen of enlarged endosomes in cultured neurons expressing Rab5 Q79L GFP , as shown by the immunostaining of its cytodomain ( Fig. 4c–f ). The luminal localization of the APP cytodomain was also found in naturally occurring enlarged endolysosomal structures, as shown by costainings with anti-EEA1, -Vps35 and -LAMP1 antibodies ( Supplementary Fig. S4b ). Importantly, immuno-EM labelling of neurons with antibodies to APP cytodomain showed gold particles associated with ILVs of multivesicular endosomes, which were also LAMP1-positive ( Fig. 4g ). 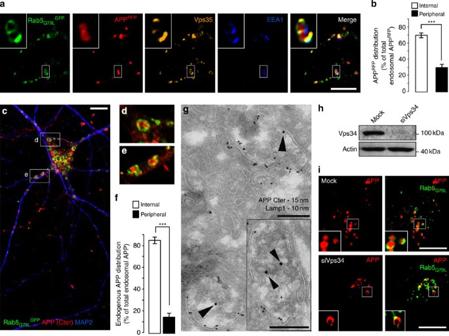Figure 4: APP is sorted into the ILVs of multivesicular endosomes. (a) Confocal analysis of HeLa cells transfected with APPRFP(red) and the dominant-positive Rab5Q79LGFPmutant (green), which was used for its ability to generate giant endosomes. The cells were fixed and labelled with anti-EEA1 (blue) and anti-Vps35 (orange) antibodies. Scale bar, 10 μm. (b) Bar diagram showing a quantification of the localization of APPRFPinside the endosomal lumen (internal) versus on the endosomal limiting membrane (peripheral), expressed as percentage of the total endosomal APPRFP. Values denote means±s.e.m. (n=20 cells from three experiments with an average quantification of 15 endosomes per cell). ***P-values<0.001 using Student’st-test. (c) Confocal analysis of mouse hippocampal neurons transfected with Rab5Q79LGFP(green) at DIV 9 and stained for endogenous APP (using the Cter antibody, red) and MAP2, a marker of the somatodendritic compartment (blue). Two insets are selected and presented in panelsdande. Scale bar, 10 μm. (d) First inset showing a magnification of the area containing enlarged endosomes presented in panelc. (e) Second inset showing a magnification of the area containing enlarged endosomes presented in panelc. (f) Bar diagram showing the quantification of the endosomal localization of endogenous APP in neurons, as in panelb. ***P-values<0.001 using Student'st-test. (g) Immunogold EM analysis of mouse hippocampal neurons at DIV 15 in ultrathin cryosections double labelled with antibodies to endogenous APP COOH-terminal domain (APP C-ter; PAG 15 nm, arrowheads), located primarily on the ILVs, and LAMP-1 (PAG 10 nm). Scale bars, 250 nm. (h) Western blot analysis of endogenous Vps34 and the loading marker actin in HeLa cells transfected with mock siRNA (mock) or siRNA against human Vps34 (siVps34) followed by transfection with APPRFPand Rab5Q79LGFP. (i) Confocal analysis of HeLa cells transfected with mock siRNA (mock, top panel) or siVps34 (bottom panel) for 72 h and then split, before transfection with APPRFPand Rab5Q79LGFP. Scale bar, 10 μm. Figure 4: APP is sorted into the ILVs of multivesicular endosomes. ( a ) Confocal analysis of HeLa cells transfected with APP RFP (red) and the dominant-positive Rab5 Q79L GFP mutant (green), which was used for its ability to generate giant endosomes. The cells were fixed and labelled with anti-EEA1 (blue) and anti-Vps35 (orange) antibodies. Scale bar, 10 μm. ( b ) Bar diagram showing a quantification of the localization of APP RFP inside the endosomal lumen (internal) versus on the endosomal limiting membrane (peripheral), expressed as percentage of the total endosomal APP RFP . Values denote means±s.e.m. ( n =20 cells from three experiments with an average quantification of 15 endosomes per cell). *** P -values<0.001 using Student’s t -test. ( c ) Confocal analysis of mouse hippocampal neurons transfected with Rab5Q79L GFP (green) at DIV 9 and stained for endogenous APP (using the Cter antibody, red) and MAP2, a marker of the somatodendritic compartment (blue). Two insets are selected and presented in panels d and e . Scale bar, 10 μm. ( d ) First inset showing a magnification of the area containing enlarged endosomes presented in panel c . ( e ) Second inset showing a magnification of the area containing enlarged endosomes presented in panel c . ( f ) Bar diagram showing the quantification of the endosomal localization of endogenous APP in neurons, as in panel b . ***P-values<0.001 using Student's t -test. ( g ) Immunogold EM analysis of mouse hippocampal neurons at DIV 15 in ultrathin cryosections double labelled with antibodies to endogenous APP COOH-terminal domain (APP C-ter; PAG 15 nm, arrowheads), located primarily on the ILVs, and LAMP-1 (PAG 10 nm). Scale bars, 250 nm. ( h ) Western blot analysis of endogenous Vps34 and the loading marker actin in HeLa cells transfected with mock siRNA (mock) or siRNA against human Vps34 (siVps34) followed by transfection with APP RFP and Rab5 Q79L GFP . ( i ) Confocal analysis of HeLa cells transfected with mock siRNA (mock, top panel) or siVps34 (bottom panel) for 72 h and then split, before transfection with APP RFP and Rab5 Q79L GFP . Scale bar, 10 μm. Full size image To determine whether the pool of APP found on ILVs originates from the plasma membrane, we performed an anti-APP ectodomain antibody (22C11) uptake experiment in HeLa cells co-expressing APP RFP and Rab5 Q79L GFP ( Supplementary Fig. S4c ). After antibody binding at 4 °C and 3 h of treatment with protein synthesis inhibitor (cycloheximide), the 22C11 immunoreactivity was mostly found at the plasma membrane, as shown by the punctate staining at the basal plane of the cells ( Supplementary Fig. S4c ). After a 15-min chase period, the 22C11 immunoreactivity was detected primarily on the limiting membrane of endosomes ( Supplementary Fig. S4d ). After 30 min, the APP RFP fluorescence (labelling the COOH-terminus) and the 22C11 fluorescence (labelling the NH 2 -terminus) converged in part in the lumen of endosomes ( Supplementary Fig. S4d ). Thus, the pool of APP that is sorted into the ILVs originates from the plasma membrane and is endocytic in nature (although a pool of cell surface-derived APP also traffics to the TGN via endosomes; see for instance, ref. 41 ). Vps34 controls the intraluminal sorting of APP in endosomes To test whether targeting of APP to ILVs is PI3P dependent, we analysed the acute effect of wortmannin, a chemical inhibitor of class I and class III PI 3-kinases. To monitor PI3P levels, HeLa cells were transfected with FYVE-FYVE GFP together with APP RFP and subjected to a 30-min treatment with 100 nM wortmannin. As expected, the drug dramatically decreased the association of FYVE-FYVE GFP with endosomes, labelled with EEA1 and Vps35 ( Supplementary Fig. S5a ). Although the localization of retromer was perturbed by this treatment, no marked phenotype was observed for APP RFP ( Supplementary Fig. S5a ). However, when this experiment was repeated after Rab5 Q79L GFP expression to visualize the endosomal lumen ( Supplementary Fig. S5b ), APP RFP was relocalized from the lumen of giant endosomes to their limiting membrane. The ratio of internal/peripheral APP RFP fluorescence in giant endosomes was quantified following wortmannin treatment in a time course-dependent fashion. APP RFP relocalization occurred very rapidly, as early as 10 min after the beginning of the treatment ( Supplementary Fig. S5b ). HeLa cells were also transfected with short interfering RNAs (siRNAs)-targeting Vps34 (siVps34) or control siRNAs (MOCK), grown for 72 h, and were then transfected with APP RFP and Rab5 Q79L GFP . The potent inhibition of Vps34 protein expression was confirmed by immunoblotting ( Fig. 4h ) and the reduction in the levels of PI3P was confirmed with a microscopic analysis of the fluorescent pattern of the FYVE-FYVE probe, either used as a glutathione S -transferase (GST) fusion for the staining of fixed cells [34] ( Supplementary Fig. S6a,b ) or as a genetically encoded GFP fusion ( Supplementary Fig. S6c ). In addition, the silencing of Vps34 produced a significant loss of membrane association of retromer component Vps35, consistent with reduced levels of PI3P ( Supplementary Fig. S6d ). As observed with wortmannin, APP RFP was mostly localized to the limiting membrane of endosomes upon siVps34 treatment ( Fig. 4i ; quantification shown in Supplementary Fig. S7c ), thus confirming the essential role of Vps34-mediated PI3P synthesis in the ILV sorting of APP. The targeting of APP to ILVs is ESCRT dependent A key player initiating the ESCRT cascade is Hrs, also known as an ESCRT0 component, which binds PI3P via a FYVE domain and ubiquitinated cargoes via a ubiquitin-interacting motif [38] , [39] . To investigate whether Hrs, like Vps34, has a role in the intraluminal sorting of APP, HeLa cells were transfected with siRNAs-targeting Hrs. Silencing Hrs ( Supplementary Fig. S7a ) produced an accumulation of APP RFP fluorescence on the limiting membrane of endosomes similar to siVps34 ( Supplementary Fig. S7b,c ). Comparable results were obtained upon silencing of ESCRT-I subunit Tsg101 and, to a lesser extent, SNX3, which has been shown to mediate the formation of ILVs in multivesicular endosomes [42] ( Supplementary Fig. S7 ). In contrast, silencing of beclin1, a major regulator of Vps34 in autophagy, did not affect the intraendosomal localization of APP ( Supplementary Fig. S7 ). Together, our data demonstrate that the Vps34/PI3P/ESCRT pathway controls the intraluminal sorting of APP. The targeting of APP to ILVs depends on its ubiquitination The signal triggering ESCRT-mediated internalization of cargoes from the limiting membrane of endosomes to ILV is ubiquitination of their cytodomain on lysine residues, either with monoubiquitins or with lysine-63-linked polyubiquitin chains [39] , [43] . We therefore tested whether endogenous APP is ubiquitinated in the brain. APP was immunoprecipitated from mouse brain extracts using anti-APP cytodomain antibodies and bound material was analysed by immunoblotting using anti-APP and -ubiquitin antibodies ( Fig. 5a ). Ubiquitin immunoreactivity was found to comigrate with APP, but not control eluate, indicating that endogenous APP is indeed ubiquitinated. 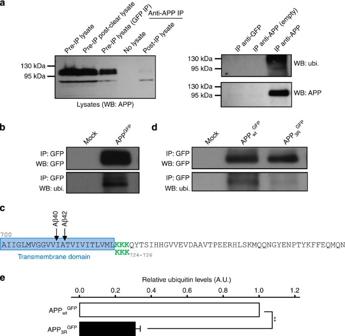Figure 5: The sorting of APP into ILVs depends on ubiquitination. (a) Mouse brain extracts were subjected to IP with an anti-APP-Cter antibody, or a control antibody (anti-GFP). Left panel: western blot analysis of the starting lysates, the post-preclearing lysate (pre-IP), the lysate post-IP with anti-GFP, the control buffer post-IP with anti-APP-Cter and the lysate post-IP with anti-APP-Cter. The immunoblot was performed with an anti-APP-Cter antibody. Right panel: western blot analysis of the immunoprecipitated material shown inausing the anti-GFP antibody (IP anti-GFP), the control IP with anti-APP-Cter without brain lysate (IP anti-APP empty) and the anti-APP-Cter antibody (IP anti-APP). The immunoblot was performed with an anti-ubiquitin antibody (top panel, ubi.), followed by stripping, and incubation with an anti-GFP antibody (bottom panel). IP, immunoprecipitated material; WB, western blot. (b) HeLa cells were transfected with APPGFPor a mock construct. Total lysates were subjected to an IP with an anti-GFP antibody. Samples were analysed by SDS–polyacrylamide gel electrophoresis (PAGE) and western blotting with an anti-ubiquitin antibody (bottom panel, ubi.), followed by stripping, and incubation with an anti-GFP antibody (top panel). IP, immunoprecipitated material; WB, western blot. (c) COOH-terminal sequence of human APP. The transmembrane domain is framed in blue, and Aβ peptide-cleavage sites are indicated with arrows. The juxtamembrane lysine residues at position 724–726 are depicted in green, and were substituted with three arginines in the APP3Rmutant. (d) HeLa cells were transfected with human APPGFP(APPWTGFP), the APP mutant (APP3RGFP), or not transfected (mock) and total lysates were prepared. After IP with an anti-GFP antibody, protein samples were analysed by SDS–PAGE and western blotting with an anti-ubiquitin antibody (bottom panel), followed by stripping, and incubation with an anti-GFP antibody (top panel). IP, immunoprecipitated material; WB, western blot. (e) Bar diagram showing the quantification of relative ubiquitin levels in APPWTand the APP3Rmutant. A.U., arbitrary units. Values denote means±s.e.m. (n=3). **P-values<0.01 using Student’st-test. Figure 5: The sorting of APP into ILVs depends on ubiquitination. ( a ) Mouse brain extracts were subjected to IP with an anti-APP-Cter antibody, or a control antibody (anti-GFP). Left panel: western blot analysis of the starting lysates, the post-preclearing lysate (pre-IP), the lysate post-IP with anti-GFP, the control buffer post-IP with anti-APP-Cter and the lysate post-IP with anti-APP-Cter. The immunoblot was performed with an anti-APP-Cter antibody. Right panel: western blot analysis of the immunoprecipitated material shown in a using the anti-GFP antibody (IP anti-GFP), the control IP with anti-APP-Cter without brain lysate (IP anti-APP empty) and the anti-APP-Cter antibody (IP anti-APP). The immunoblot was performed with an anti-ubiquitin antibody (top panel, ubi. ), followed by stripping, and incubation with an anti-GFP antibody (bottom panel). IP, immunoprecipitated material; WB, western blot. ( b ) HeLa cells were transfected with APP GFP or a mock construct. Total lysates were subjected to an IP with an anti-GFP antibody. Samples were analysed by SDS–polyacrylamide gel electrophoresis (PAGE) and western blotting with an anti-ubiquitin antibody (bottom panel, ubi. ), followed by stripping, and incubation with an anti-GFP antibody (top panel). IP, immunoprecipitated material; WB, western blot. ( c ) COOH-terminal sequence of human APP. The transmembrane domain is framed in blue, and Aβ peptide-cleavage sites are indicated with arrows. The juxtamembrane lysine residues at position 724–726 are depicted in green, and were substituted with three arginines in the APP 3R mutant. ( d ) HeLa cells were transfected with human APP GFP (APP WT GFP ), the APP mutant (APP 3R GFP ), or not transfected (mock) and total lysates were prepared. After IP with an anti-GFP antibody, protein samples were analysed by SDS–PAGE and western blotting with an anti-ubiquitin antibody (bottom panel), followed by stripping, and incubation with an anti-GFP antibody (top panel). IP, immunoprecipitated material; WB, western blot. ( e ) Bar diagram showing the quantification of relative ubiquitin levels in APP WT and the APP 3R mutant. A.U., arbitrary units. Values denote means±s.e.m. ( n =3). ** P -values<0.01 using Student’s t -test. Full size image To determine the main ubiquitination sites relevant for ILV sorting, HeLa cells were transfected with APP GFP and lysates were subjected to immunoprecipitation (IP) using anti-GFP antibodies. Immunoblotting of the immunoprecipitated material with an anti-ubiquitin antibody revealed that APP GFP is also ubiquitinated ( Fig. 5b ), similar to endogenous APP. A stretch of three lysines located in the cytoplasmic juxtamembrane region on positions 724–726 of human APP were good candidate ubiquitination sites (green residues in Fig. 5c ), based on evidence from others indicating that lysines in the juxtamembrane region of proteins can be ubiquitinated [44] and the recent finding that lysine 726 ubiquitination is relevant for proteasomal degradation of APP under conditions of overexpression of F box factor FBL2 [45] . To determine the role of these lysines, an APP mutant in which lysines 724–726 were substituted with arginines (referred to as APP 3R GFP ) was expressed in HeLa cells and showed a dramatic reduction in the ubiquitin signal relative to the control ( Fig. 5d,e ). To test whether ubiquitination of these lysine residues is critical for ILV sorting, we expressed APP 3R GFP and Rab5 Q79L myc and examined the targeting of mutant APP to ILVs in giant endosomes. We found that APP 3R GFP displayed a predominant association with the limiting membrane of endosomes at the expense of luminal localization ( Fig. 6a,b ). When expressed in hippocampal neurons alongside Rab5 Q79L GFP , APP 3R also exhibited decreased targeting to the lumen of enlarged endosomes relative to APP WT ( Fig. 6c,d ), although the missorting was not as striking as that observed in HeLa cells. Importantly, treatment with γ-secretase inhibitor (compound XXI) was applied in these experiments to enhance and better visualize the endosomal pool of APP, which otherwise undergoes significant processing by the secretase (see below). Together, our results demonstrate that ubiquitination of the cytodomain of APP on one or more of lysines 724–726 is important for the intraluminal sorting of APP through the Vps34/PI3P/ESCRT pathway. 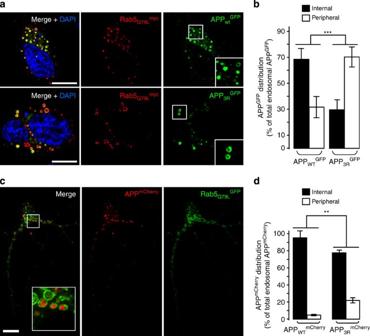Figure 6: Blocking the intraluminal sorting of APP enhances its amyloidogenic processing. (a) Confocal analysis of HeLa cells transfected with Rab5Q79Lmycand APPWTGFP(top panel) or APP3RGFP(middle panel). Cells were labelled with an anti-myc antibody (red) and counterstained with 4',6-diamidino-2-phenylindole (DAPI; blue). Scale bar, 10 μm. (b) Bar diagram showing the quantification of the endosomal distribution of human APPGFPexpressed as percentage of total endosomal APPGFP: internal=inside endosomal lumen, peripheral=limiting membrane of the endosomes. Values denote means±s.e.m. (for each construct,n=18 cells from three experiments with an average quantification of 15 endosomes per cell). ***P-values<0.001 using Student’st-test. (c) Confocal analysis of mouse hippocampal neurons transfected at DIV 9 with Rab5Q79LGFPand APPWTmCherryand fixed after a 24-h treatment with γ-secretase inhibitor XXI. Scale bar, 10 μm. The inset shows APP-containing endosomes. (d) Bar diagram showing the quantification of the endosomal distribution of human APPWTmCherryand APP3RmCherryin hippocampal neurons processed, as described inc. The APPmCherrydistribution is expressed as percentage of total endosomal APPmCherry: internal=inside endosomal lumen, peripheral=limiting membrane of the endosomes. Values denote means±s.e.m. (n=45 and 18 cells for APPWTmCherryand APP3RmCherry, respectively, from three experiments with an average quantification of 20 endosomes per cell). **P-values<0.01 using Student’st-test. Figure 6: Blocking the intraluminal sorting of APP enhances its amyloidogenic processing. ( a ) Confocal analysis of HeLa cells transfected with Rab5 Q79L myc and APP WT GFP (top panel) or APP 3R GFP (middle panel). Cells were labelled with an anti-myc antibody (red) and counterstained with 4',6-diamidino-2-phenylindole (DAPI; blue). Scale bar, 10 μm. ( b ) Bar diagram showing the quantification of the endosomal distribution of human APP GFP expressed as percentage of total endosomal APP GFP : internal=inside endosomal lumen, peripheral=limiting membrane of the endosomes. Values denote means±s.e.m. (for each construct, n =18 cells from three experiments with an average quantification of 15 endosomes per cell). *** P -values<0.001 using Student’s t -test. ( c ) Confocal analysis of mouse hippocampal neurons transfected at DIV 9 with Rab5 Q79L GFP and APP WT mCherry and fixed after a 24-h treatment with γ-secretase inhibitor XXI. Scale bar, 10 μm. The inset shows APP-containing endosomes. ( d ) Bar diagram showing the quantification of the endosomal distribution of human APP WT mCherry and APP 3R mCherry in hippocampal neurons processed, as described in c . The APP mCherry distribution is expressed as percentage of total endosomal APP mCherry : internal=inside endosomal lumen, peripheral=limiting membrane of the endosomes. Values denote means±s.e.m. ( n =45 and 18 cells for APP WT mCherry and APP 3R mCherry , respectively, from three experiments with an average quantification of 20 endosomes per cell). ** P -values<0.01 using Student’s t -test. Full size image The APP3R mutant shows altered sorting in neurons Silencing Vps34 produced a dramatic loss of endogenous APP fluorescence in neuronal endosomes, a phenotype rescued by γ-secretase inhibitor treatment. If a key function of PI3P is to promote ILV sorting of APP into multivesicular endosomes through ESCRT, the traffic pattern of APP 3R may phenocopy that of wild-type APP obtained upon Vps34 silencing. As hypothesized, the association of APP 3R with neuronal endosomes positive for EEA1 ( Fig. 7 ) or Vps35/retromer ( Supplementary Fig. S8 ) was dramatically reduced, whereas that with the GM130-positive Golgi compartment was slightly enhanced ( Supplementary Fig. S9 ) relative to APP WT . As seen with the Vps34 knockdown, treatment of neurons with the γ-secretase inhibitor restored the normal distribution of APP 3R ( Fig. 7 , Supplementary Figs S8 and S9 ), although within endosomes, the APP 3R mutant was preferentially localized on the limiting membrane ( Fig. 6c,d ). 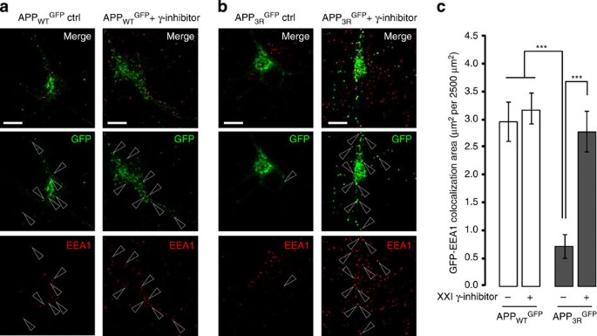Figure 7: Decreasing the ubiquitination of APP alters its subcellular localization in primary neurons. (a,b) Mouse neurons were transfected with human APPWTGFP(a) and APP3RGFP(b) plasmids at DIV 9. After 24 h expression in the presence (right panels) or absence (left panels) of γ-secretase inhibitor compound XXI, neurons were fixed, stained for EEA1 (red channel) and imaged with confocal microscopy. Scale bar, 10 μm. Arrowheads indicate structures where APPGFPand EEA1 colocalize. (c) Bar diagram showing the amount of colocalization between GFP and EEA1 per 2500 μm2of image cell surface area following expression of APPWTGFPand APP3RGFPin cultured neurons, in the presence or absence of γ-secretase inhibitor XXI. Results are shown as means±s.e.m. (APPWTGFP,n=30 and APP3RGFP,n=20). ***P-values<0.001 using Student’st-test. Figure 7: Decreasing the ubiquitination of APP alters its subcellular localization in primary neurons. ( a , b ) Mouse neurons were transfected with human APP WT GFP ( a ) and APP 3R GFP ( b ) plasmids at DIV 9. After 24 h expression in the presence (right panels) or absence (left panels) of γ-secretase inhibitor compound XXI, neurons were fixed, stained for EEA1 (red channel) and imaged with confocal microscopy. Scale bar, 10 μm. Arrowheads indicate structures where APP GFP and EEA1 colocalize. ( c ) Bar diagram showing the amount of colocalization between GFP and EEA1 per 2500 μm 2 of image cell surface area following expression of APP WT GFP and APP 3R GFP in cultured neurons, in the presence or absence of γ-secretase inhibitor XXI. Results are shown as means±s.e.m. (APP WT GFP , n =30 and APP 3R GFP , n =20). *** P -values<0.001 using Student’s t -test. Full size image Inhibiting ILV sorting of APP enhances Aβ levels Our data suggest that APP 3R is more extensively processed through the amyloidogenic pathway in endosomes, similar to endogenous APP in the Vps34 knockdown. We thus examined the impact of the 3R mutation on the metabolism of APP expressed exogenously with lentivirus in primary neurons (in the absence of Rab5 Q79L expression). Constructs were comparably expressed, based on the lack of differences found for FL-APP WT and APP 3R ( Fig. 8a ). Similar to the Vps34 knockdown, sAPP-α levels were unchanged ( Fig. 8b ), whereas a trend for an increase in sAPP-β was found for the APP 3R mutant ( Fig. 8c ). Consistent with this trend, expression of APP 3R caused an ~50% increase in Aβ40, although surprisingly Aβ42 levels were unchanged ( Fig. 8d ). Together, these data indicate that mutations that decrease the intraluminal sorting of APP in endosomes promote the generation of Aβ. 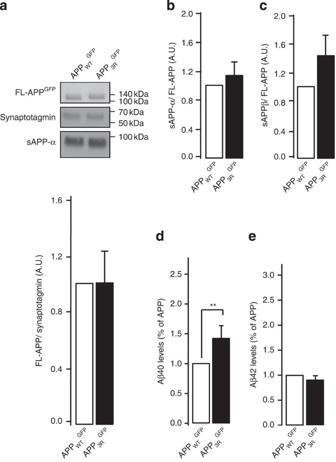Figure 8: Expression of the APP3R mutant leads to an increase in secreted Aβ. (a,b) Mouse neurons were infected with lentiviruses expressing human APPWTGFPand APP3RGFPat DIV 7. At DIV 14, secreted APP metabolite sAPP-α was analysed by SDS–polyacrylamide gel electrophoresis and western blot (a,b), whereas secreted APP metabolite sAPP-β was measured by enzyme-linked immunosorbent assay (ELISA) of culture media (c). Synaptotagmin was used as an equal loading marker. The graphs show the quantification of full-length APP normalized to synaptotagmin (a) and the quantification of metabolites sAPP-α (b) and sAPP-β levels (c) as a ratio of metabolite/full-length APPGFP. Values denote means±s.e.m. (n=8). (d,e) Bar diagram showing the quantification of human Aβ40 (d) and Aβ42 (e) peptide levels measured by ELISA in neuronal media after infection of neurons with lentiviruses expressing human APPWTGFPor APP3RGFP. Aβ levels were normalized to the cell lysate total protein and results are expressed as percentage of APPWTGFP. Values denote means±s.e.m. (n=13). **P-values<0.01 using Student’st-test. Figure 8: Expression of the APP3R mutant leads to an increase in secreted Aβ. ( a , b ) Mouse neurons were infected with lentiviruses expressing human APP WT GFP and APP 3R GFP at DIV 7. At DIV 14, secreted APP metabolite sAPP-α was analysed by SDS–polyacrylamide gel electrophoresis and western blot ( a , b ), whereas secreted APP metabolite sAPP-β was measured by enzyme-linked immunosorbent assay (ELISA) of culture media ( c ). Synaptotagmin was used as an equal loading marker. The graphs show the quantification of full-length APP normalized to synaptotagmin ( a ) and the quantification of metabolites sAPP-α ( b ) and sAPP-β levels ( c ) as a ratio of metabolite/full-length APP GFP . Values denote means±s.e.m. ( n =8). ( d , e ) Bar diagram showing the quantification of human Aβ40 ( d ) and Aβ42 ( e ) peptide levels measured by ELISA in neuronal media after infection of neurons with lentiviruses expressing human APP WT GFP or APP 3R GFP . Aβ levels were normalized to the cell lysate total protein and results are expressed as percentage of APP WT GFP . Values denote means±s.e.m. ( n =13). ** P -values<0.01 using Student’s t -test. Full size image Cell biological observations combined with results from expression and genetic profiling have suggested that defects in endosomal sorting and trafficking have a pathogenic role in AD [1] , [4] , [5] . Together with studies suggesting that amyloidogenic processing of APP predominantly occurs in endosomes, these reports indicate that these organelles are critical players in AD pathogenesis. Our study strongly supports this hypothesis by identifying a molecular defect, namely, a selective deficiency in PI3P, in affected brain regions from patients with LOAD as well as in the forebrain of mouse models of FAD. Remarkably, the deficiency of PI3P is the only lipid change common to both human and mouse brains affected by AD out of ~330 lipid species examined. As the PI3P deficiency does not correlate with the extent of neuronal death or AD pathology in AD-affected regions, it is unlikely to merely stem from neurodegeneration, although it may also reflect changes occurring in glial cells. PI3P controls fundamental aspects of endosomal membrane dynamics [26] , [27] , [39] . In addition, PI3P regulates macroautophagy, which mediates via an interplay with endolysosomal compartments the clearance of defective organelles and intracellular aggregates, and has also been implicated in AD [29] , [36] . Although a deficiency of PI3P in AD may theoretically cause any of the abovementioned PI3P-dependent processes to function suboptimally, our study provides strong evidence that it affects endosome dynamics as well as the sorting and processing of APP, all of which are believed to have a role in AD pathogenesis. Indeed, modelling the PI3P deficiency by silencing Vps34, the main source of PI3P, produces endosomal enlargement, a perturbation of APP trafficking as well as increased production of Aβ. Interestingly, these phenotypes are partially shared in common by instances in which Rab5 is overexpressed [5] , [12] . However, the link between PI3P deficiency and Rab5 hyperactivation identified in LOAD is unclear, as Rab5 is known to activate Vps34 [46] . We speculate that Rab5 hyperactivation may be compensating for the PI3P deficiency, although these phenomena may not be directly related. Our cell culture studies indicate that APP is sorted and trafficked via ESCRT, and together with previous studies implicating the retromer pathway suggest a general mechanism for how PI3P deficiency observed in the disease can lead to APP missorting. In common with recent studies [45] , [47] , we found that APP is ubiquitinated on cytoplasmic lysine residues. However, extending on these observations, we found that ubiquitination, which we document also for the endogenous protein in the brain, mediates targeting of an endocytic pool of APP to ILVs via ESCRT, rather than to proteasomal degradation. Indeed, silencing key ESCRT components, such as Hrs and Tsg101, leads to an accumulation of APP on the limiting membrane of endosomes in HeLa cells, which express low levels of BACE1. Furthermore, substituting the lysine residues with arginines dramatically impairs ubiquitination of APP and also causes a shift of its localization to the limiting membrane of endosomes. Remarkably, ILV missorting correlates with elevation of Aβ secretion in neurons, although the pattern of secreted Aβ species varies depending on the specific manipulation; while Vps34 silencing causes an increase in both Aβ40 and 42, the APP 3R mutant causes a differential elevation in Aβ40. This is consistent with the idea that the PI3P deficiency may also cause defects in APP trafficking and processing independently of those produced by reduced ESCRT-dependent sorting into ILV. In this respect, a key effect of PI3P deficiency may be to cause a dysfunction of retromer, whose knockdown phenocopies the increase in Aβ40 and 42 levels in neurons [23] . Interestingly, the selective increase in Aβ40 observed with the APP 3R mutant may paradoxically confer protection against amyloidogenesis in vivo , based on the ability of this shorter peptide to counteract the aggregate-inducing property of Aβ42 (ref. 48 ). Regardless, our data suggest that Aβ generation predominantly occurs on the limiting membrane of neuronal endosomes, perhaps reflecting the presence there of highly active pools of BACE1 and/or presenilin. This is supported by our experiments showing that γ-secretase inhibitors restore an endosomal pool of APP that is otherwise drastically diminished by the silencing of Vps34 or the 3R mutation of APP. We note that some studies in non-neuronal cell lines have reported experimental manipulations that enhance the Golgi association of APP (at the expense of endosomes) as well as its amyloidogenic processing (see for instance, ref. 35 ). The use of γ-secretase inhibitors in those instances should help to resolve whether the loss of endosomal pool reflects enhanced processing in those organelles rather than a bona fide accumulation of APP in the Golgi compartment. We also note that a recent APP overexpression study conducted in non-neuronal cells reported that silencing various ‘early’ ESCRT components (for example, Hrs, Tsg101) causes a retention of APP in endosomes and a decrease of Aβ40 release. Conversely, silencing ‘late’ ESCRT components (for example, CHMP6, Vps4) causes enhanced targeting of APP to the TGN and an increase in Aβ40 release [41] . Future work should address whether these experimental manipulations produce similar results in neurons. Overall, our study and work from others suggest that the pathogenesis of AD, and LOAD in particular, is linked to the dysfunction of a number of genes involved in trafficking pathways identified in yeast as ‘vacuolar protein sorting’ (for example, Vps34 and beclin1/Vps30 (PI3K), Hrs/Vps27 and Tsg101/Vps23 (ESCRT), Vps26/29/35 (retromer), SorLa/SorCs1 (Vps10-like proteins)) [22] , [28] , [49] . The identification of PI3P deficiency in affected brain regions of individuals with LOAD not only provides a potential mechanism explaining AD-associated endosomal anomalies and aberrant APP metabolism but also defects in autophagy [28] , [36] , which may reduce clearance of tau aggregates [50] . The precise genetic and/or environmental factors responsible for PI3P deficiency in FAD and LOAD are unknown, although we speculate they may affect the function of Vps34 complexes, perhaps in combination with that of alternate pathways controlling PI3P levels. Finally, besides clarifying basic mechanisms of APP biology, our results may have clinical implications. In particular, our data suggest that as an enzyme that regulates PI3P levels, Vps34, as well as other lipid enzymes controlling PI3P levels through dephosphorylation mechanisms (for example, myotubularins) may be novel targets for drug discovery in attempting to improve APP missorting characteristic of LOAD. In this respect, targeting the metabolism of phosphoinositides, and more generally phospholipids, is emerging as a promising new avenue for AD therapy [31] , [32] , [51] , [52] , [53] . As recent studies have implicated defects either in lipid metabolism or in endosomal sorting in AD, our work establishes an important link between these two intracellular processes, and this converging view also provides a focus for developing novel therapeutic targets and agents. Human and mouse brain tissue Frozen post-mortem brain tissue samples were obtained from the New York Brain Bank at Columbia University Medical Center, and are described previously [33] . Three different brain regions were sampled: PFC, ERC and CRB. The diagnostic criteria for AD were based on the presence of neurofibrillary tangles, senile plaques and dementia. Wild-type, PS1, APP and PS1-APP mice, which were aged between 9 and 11.5 months, were described previously [33] . All mice were killed by cervical dislocation, the forebrain was dissected immediately and frozen in liquid nitrogen before storage at −80°C. Cell transfection and lentivirus production HeLa and HEK-293T cells were grown at 37 °C in a 5% CO 2 incubator in MEM and DMEM, respectively (Invitrogen). HeLa cells were transiently transfected using Fugene-6 (Roche Diagnostics) or Lipofectamine 2000 (Invitrogen) for complementary DNA (from 24 to 48 h) and siRNA (72 h), respectively. Hippocampal cultures were obtained from P0 mice. Neurons were plated on poly- L -lysine-coated coverslips or six-well plates, and were incubated with Neurobasal media (Invitrogen) with 10% fetal bovine serum. After 5 h, neurons were transferred into serum-free medium supplemented with B27 (Invitrogen) and cultured for 9–12 days in vitro (DIV). In some experiments, neurons cultured for 8–9 days were transfected for 60 min with 2 μl of Lipofectamine 2000 combined with 1 μg of DNA, washed and incubated for 24 h (APP WT GFP , APP 3R GFP ) or 4 days (shRNA) before immunofluorescence analysis. In other experiments, neurons were infected with shRNA lentivirus after 7 days in culture, and were cultured up to 14 days. Lentiviruses were generated by transfecting lentiviral vectors (APP WT GFP , APP 3R GFP ) or a mix of equal amounts of shVPS34-1 and shVPS34-2 into HEK-293T cells using lipofectamine LTX (Invitrogen). A pPACK-H1 packaging mix (System Biosciences) was added to the transfection reagents according to the manufacturer’s instructions. The medium was collected 48 and 72 h after transfection, passed through a 45-nm filter and applied at 1:4 ratio to media. Antibodies and reagents Antibodies were obtained from the following sources: rabbit polyclonal antibodies to Vps34 (Cell Signaling), APP (Calbiochem), sAPP-α and giantin (Covance), APP C-terminal fragments (APP-Cter; Invitrogen), LAMP1 and SNX3 (Abcam), red fluorescent protein (Rockland) and Hrs (a kind gift from G. Cesareni, University of Tor Vergata, Rome, Italy), a goat polyclonal antibody to Vps35 (Abcam), mouse monoclonal antibodies (mAbs) to actin (Novus), Tsg101 (Abcam), beta amyloid 1-42 12F4 (Covance), sAPP-α clone m3.2 (a kind gift from P. Matthews, Nathan Kline Institute, NY, USA), APP N-terminus A4 22C11 (Millipore), Rab5, Rab7 and Synaptotagmin1 (Synaptic Systems), GAPDH (EnCor Biotech), GFP (Roche Diagnostics), Myc 9E10 (Invitrogen), EEA1 and GM130 (BD Transduction Laboratories), ubiquitin P4D1 (Santa Cruz) and LC3 4E12 (MBL), and a rat polyclonal antibody to LAMP1 (BD Pharmingen). Peroxidase-conjugated secondary antibodies were from Bio-Rad and fluorescent secondary antibodies (Alexa and Cyanin) were from Jackson Immunoresearch and Invitrogen. PI3-kinase activity was blocked with 100 nM wortmannin (Invitrogen). To prevent autophagosome clearance, cells were treated with 50 nM bafilomycin A1 (Waco) for 1 h. γ-secretase was blocked for 24 h with 10 μM γ-secretase Inhibitor XXI, Compound E (both from Calbiochem). Plasmids and RNA interference Plasmids were kindly provided by the following sources: human Rab5 Q79L GFP (M. Zerial, Dresden, Germany), Rab5 Q79L myc (J. Gruenberg, Geneva, Switzerland), FYVE-FYVE GST and FYVE-FYVE GFP (H. Stenmark, Oslo, Norway), human Vps34 RFP (N. Ktistakis, Cambridge, UK) and monomeric RFP (Roger Tsien, UCSD, California, USA). The APP GFP and APP MYC plasmids were constructed by excising the APP cDNA from APP RFP (derived from NM_201414.2) with Sal I/ Hin dIII, and subcloning it into pEGFP-N3 (Clonetech) and pCMV5A (Stratagene). APP 3R GFP was generated by quick mutagenesis on APP GFP with the following primer and its antisense: 5′-CACCTTGGTGATGCTGAgGAgGAgACAGTACACATCCATTC-3′. Human APP GFP and APP 3R GFP lentiviruses were constructed by excising APP GFP and APP 3R GFP , respectively, from pEGFP-N3 with Nhe I/ Not I and ligating the cDNAs into pCDH-CMV-MCSr (System Biosciences). Human APP mCherry and APP 3R mCherry were constructed by Sal I/ Not I replacement of GFP in APP GFP , and APP 3R GFP with a mCherry including Sal I/ Not I overhangs. For RNA interference in HeLa cells, we used an equal mix of the following predesigned human siRNA sequences (Qiagen): Vps34 (SI00040950/SI00040971), Hrs (SI00288239/SI02659650), Tsg101 (SI02655184/SI02664522), SNX3 (S104309704/S103150280) and Beclin1 (S100055573/S100055580). Mouse Vps34-shRNA lentivectors were generated with the pSIH-H1 shRNA vector from System Biosciences. The control was pSIH1-H1-copGFP Luciferase shRNA, and the Vps34-shRNA targets were as follow: mVps34-1 shRNA, 5′-GTGGAGAGCAAACACCACAAGCTTGCTCG-3′; mVps34-2 shRNA, 5′-CCTGACCTGCCCAGGAATGCCCAAGTGGC-3′. Lipid analysis Phosphoinositide-enriched lipid fractions were extracted from frozen brain tissue samples (80–120 mg), deacylated and analysed by anion-exchange high-performance liquid chromatography with suppressed conductivity detection as described [30] , [31] but with slight modification to the KOH gradient profile to better resolve PI4P and PI3P elution ( Supplementary Fig. S1 ). Specifically, the elution was carried out in five stages: (1) a gradient change of 1.5–4 mM KOH from the injection time to 7 min after injection, (2) 4–16 mM from 7–12 min after injection, (3) 16–25.75 mM from 12–35 min after injection, (4) 25.75–86 mM from 35–60 min after injection and (5) 5 min isoelectric elution with 86 mM KOH. A portion of the same tissues used above was subjected to lipidomics analysis using LC–MS, as previously described [33] . Fluorescence microscopy Cells were fixed with 4% paraformaldehyde for 30 min and permeabilized with 0.05% saponin together with primary antibodies in PBS supplemented with 5% fetal calf serum. For the anti-APP-Cter staining, neurons were permeabilized with 0.2% Triton X-100 for 10 min. For other stainings, neurons were permeabilized with 0.01% digitonin. For the labelling of PI3P with FYVE-FYVE GST , cells were fixed and incubated for 1 h with purified FYVE-FYVE GST recombinant protein (20 μg ml −1 final concentration), washed with PBS and labelled with a FITC-conjugated anti-GST antibody (Abcam). Coverslips were mounted in mowiol or DAPI-mowiol (Sigma) or ProLong Gold (Invitrogen). Images were acquired by confocal laser scanning microscopy (Zeiss LSM 700 and 510) and analysed with Zeiss Zen and imageJ softwares. Ultracryomicrotomy and immunogold labelling Hippocampal neurons at 15 DIV were fixed with a mixture of 2% (wt/vol) PFA and 0.125% (wt/vol) glutaraldehyde in 0.1 M PBS, pH 7.4. Cell pellets were washed with PBS, embedded in 10% (wt/vol) gelatin and infused in 2.3 M sucrose [54] . Mounted gelatin blocks were frozen in liquid nitrogen and ultrathin sections were prepared with an EM UC6 ultracryomicrotome (Leica). Ultrathin cryosections were collected with 2% (vol/vol) methylcellulose, 2.3 M sucrose and single or double immunogold labelled with antibodies and protein A coupled to 5 or 10 nm gold (PAG5 and PAG10; obtained from the Cell Microscopy Center of Utrecht University Hospital, Netherlands), as reported previously [54] . Sections were observed under Philips CM-12 electron microscope (FEI; Eindhoven, The Netherlands) and photographed with a Gatan (4 k × 2.7 k) digital camera (Gatan, Inc., Pleasanton, CA, USA). Protein biochemistry and immunoblotting Total endosome fractions, comprising both early and late endosomal membranes, were generated as previously described [55] . To detect ubiquitinated APP, HeLa cells were transiently transfected with human APP WT GFP or APP 3R GFP and then lysed for 30 min at 4 °C in IP buffer (0.5% NP-40, 500 mM Tris–HCl, pH 7.4, 20 mM EDTA, 10 mM NaF, 30 mM sodium pyrophosphate decahydrate, 2 mM benzamidine, 1 mM phenylmethanesulfonylfluoride, 1 mM N -ethyl-maleimide and a cocktail of protease inhibitors), centrifuged for 3 min at 2000 g , and supernatants were precleared with protein G-coupled beads (Invitrogen) before an incubation for 2 h at 4 °C with protein G-coupled beads and 2 μg anti-GFP mAb. For IP using mouse brain, tissue was collected and homogenized on ice with a Dounce homogenizer in IP buffer. After 30 min at 4 °C, homogenates were centrifugated at 13000 g for 5 min. After preclearing, 500 μl of lysate were incubated for 2 h at 4 °C with protein G-coupled beads and 10 μg anti-APP-Cter polyclonal antibody or 3 μg anti-GFP mAb (as a control). After washing the beads with IP buffer, proteins were eluated, separated on a Bis–Tris gel (Invitrogen) and transferred by a semi-dry method on a nitrocellulose membrane. The latter was then probed sequentially with an anti-ubiquitin and anti-GFP antibody (after stripping). Quantification was made with Image J or the LAS4000 softwares. For all other immunoblots, cells were lysed for 30 min at 4 °C in RIPA buffer with protease and phosphatase inhibitor cocktails, centrifuged for 15 min at 13000 g , and proteins in the supernatant were processed for SDS–PAGE and immunoblotting. Please see Supplementary Fig. S10 for full scans of imunoblots. Enzyme-linked immunosorbent assays Murine Aβ1-40 and Aβ1-42 were measured from the medium of hippocampal cultures infected with a mix of shVps34 lentiviruses to monitor endogenous APP processing, and human Aβ1-40, Aβ1-42 and sAPP-β were quantified from the media of neurons infected with human APP-WT-GFP or APP3R-GFP lentiviruses. The enzyme-linked immunosorbent assay kits were from Invitrogen (Aβ) and Covance (sAPP-β), and the experiments were performed according to the manufacturer’s instructions. Briefly, neurons were infected 7 days after plating, and the medium was collected 7 days after infection and supplemented with 0.25 mg ml −1 Pefabloc SC 4-(2-Aminoethyl) benzenesulfonyl fluoride hydrochloride (Fluka Analytical). Each sample was then measured in duplicates. Statistics Statistical analysis was performed using the Student’s t -test (for the comparison of two averages), the one-sample t -test (for the comparison of one average to a normalized value where variability is lost), the one-way analysis of variance test with post hoc least significant difference or Tukey test (for the comparison of three or more averages). In Fig. 1a , a one-tailed Student’s t -test was exceptionally used for the PI(4,5)P 2 data, based on predictions from previously published work showing Aβ disrupts the metabolism of this lipid [31] . How to cite this article: Morel, E. et al . Phosphatidylinositol-3-phosphate regulates sorting and processing of amyloid precursor protein through the endosomal system. Nat. Commun. 4:3250 doi: 10.1038/ncomms3250 (2013).